Alkyne–Alkene [2 + 2] cycloaddition based on visible light photocatalysis UV-activated alkyne–alkene [2 + 2] cycloaddition has served as an important tool to access cyclobutenes. Although broadly adopted, the limitations with UV light as an energy source prompted us to explore an alternative method. Here we report alkyne–alkene [2 + 2] cycloaddition based on visible light photocatalysis allowing the synthesis of diverse cyclobutenes and 1,3-dienes via inter- and intramolecular reactions. Extensive mechanistic studies suggest that the localized spin densities at sp 2 carbons of alkenes account for the productive sensitization of alkenes despite their similar triplet levels of alkenes and alkynes. Moreover, the efficient formation of 1,3-dienes via tandem triplet activation of the resulting cyclobutenes is observed when intramolecular enyne cycloaddition is performed, which may serve as a complementary means to the Ru(II)-catalyzed enyne metathesis. In addition, the utility of the [2 + 2] cycloaddition has been demonstrated by several synthetic transformations including synthesis of various extended π-systems. The synthesis of cyclobutenes has drawn much attention from the synthetic community owing to their versatility as synthetic intermediates and their presence in complex natural products [1] . Since thermal [2 + 2] cycloaddition of alkynes with alkenes is a thermally forbidden process, the synthesis of cyclobutenes has been developed primarily based on direct excitation by UV light (Fig. 1a ) [2] , [3] , [4] , [5] , [6] . Recently, a chiral UV sensitizer has been reported for enantioselective synthesis of cyclobutenes [7] . On the other hand, various alternative methods including Lewis acid- [8] , [9] , [10] , [11] and transition metal- [12] , [13] , [14] , [15] , [16] catalyzed syntheses of cyclobutenes have been developed. However, the requirement of specific functional groups on the substrates for activation remains as limitation. Fig. 1: Synthesis of 4-membered ring carbocycles. a Previous works for the synthesis of cyclobutenes, cyclobutanes, and 1,3-dienes. b This work for the synthesis of cyclobutenes and 1,3-dienes via visible light EnT photocatalysis. Full size image The past decade has seen a surge of developments in visible-light photocatalysis [17] , [18] , [19] , [20] . A number of elegant syntheses have been reported based on electron transfer (ET) photoredox processes [21] , [22] , [23] , [24] , [25] , [26] . Meanwhile, energy transfer (EnT) processes have drawn attention as an alternative visible-light photocatalysis in an increasing number of transformations [27] , [28] , [29] . For example, synthesis of N-heterocycles via sensitization of azido compounds [30] , [31] , [32] , [33] , [34] , [35] and isomerization of alkenes [36] , [37] , [38] have been described. Also, alkene–alkene [2 + 2] cycloaddition for the synthesis of cyclobutanes in inter- and intramolecular fashion based on the EnT process has been reported [39] , [40] , [41] , [42] , [43] , [44] , [45] , [46] . Meanwhile, only a limited number of studies on the alkyne–alkene reactions with visible light photocatalysis have been reported. Very recently, Glorius [47] and Maestri [48] groups described novel alkyne–alkene reactions under visible light photocatalysis. 1,3-Dienes are a valuable synthetic moiety that are found in a wide variety of transformations. Intense research efforts have been made to develop efficient synthesis. For example, a number of elegant synthesis 1,3-dienes based on transition metal-catalysis including gold [49] , [50] , [51] , palladium [52] , [53] , and platinum [54] , [55] . Also, enyne metathesis with Grubbs catalysts has proven to be an efficient method for the synthesis of various 1,3-dienes [56] , [57] . Meanwhile, direct access to 1,3-dienes from enynes based on visible-light photocatalysis would offer a complementary route to enyne metathesis. Here we report the visible light EnT-based alkyne–alkene [2 + 2] cycloaddition, which displays an intriguing dichotomy in reactivity with respect to the types of substrates (Fig. 1b ). Whereas the intermolecular reaction affords cyclobutenes, the formation of 1,3-dienes in the case of intramolecular reaction is remarkable. 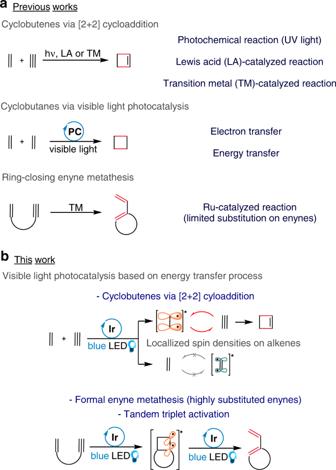Fig. 1: Synthesis of 4-membered ring carbocycles. aPrevious works for the synthesis of cyclobutenes, cyclobutanes, and 1,3-dienes.bThis work for the synthesis of cyclobutenes and 1,3-dienes via visible light EnT photocatalysis. Reaction optimization We began the screening with various photocatalysts under visible-light irradiation by employing di( p -tolyl)acetylene 1a and N -methylmaleimide 2a as the coupling partners (see Supplementary Table 1 ). It turned out that the use of 2.5 mol% Ir[dF(CF 3 )ppy] 2 (dtbbpy)PF 6 ( PC I ) was optimal to afford 3aa in 83% yield. Moreover, the cycloaddition proceeded with higher yields in nonpolar solvents under diluted concentration (CH 2 Cl 2 in 0.05 M). To confirm that the reaction is driven by photocatalysis, control reactions were performed, in which no reaction was observed in the absence of light or a catalyst. At this juncture, we were prompted to investigate the underlying factors governing the reactivity of the catalysts observed during the screening (Table 1 ). To distinguish the two plausible reaction pathways, ET and EnT, the reduction potential ( E p/2 red = −1.16 V vs. SCE) and triplet energy (55.9 kcal/mol) of N -methylmaleimide 2a were compared with those of the catalysts. A clear correlation was observed between the yields of the cycloadduct and the triplet energies of the catalysts, while their reduction potentials are inconsistent with the conversions of the reaction. For example, PC I , which has the highest triplet energy (60.8 kcal/mol), turned out to be the most efficient for cycloaddition, however, its reduction potential ( E 1/2 (M*/M + ) = −0.89 V vs. SCE) is insufficient for the reduction of 2a . On the other hand, a trace conversion was observed with the catalyst PC VI , which has a slightly higher reduction potential ( E 1/2 (M*/M + ) = −0.96 V vs. SCE) but much lower triplet energy (49.2 kcal/mol) than that of 2a . Likewise, the same trend was observed for alkyne 1a ( E p/2 red = −2.5 V, E p/2 ox = +1.59 V vs. SCE and E T = 56.7 kcal/mol), in which the yields showed good correlation with the triplet energies rather than the redox potentials of the catalysts. These observations led us to propose that EnT process is in operation for the alkyne–alkene [2 + 2] cycloaddition, although it remains unclear which counterpart between alkenes and alkynes undergoes productive triplet excitation. Table 1 Triplet energies and redox potentials of photocatalysts a . Full size table Substrate scope With the optimized conditions in hand, we investigated the scope of the intermolecular reaction. First, we examined the steric and electronic influences of substituted diarylalkynes by reacting with N -methylmaleimide 2a . It was found that both electron-rich and deficient alkynes were well tolerated (Fig. 2 , 3aa–3ha ). The utility of heterocycles in bioactive compounds prompted us to examine pyridine- and pyrazine-substituted alkynes [58] . We were gratified to find that these heterocyclic substrates reacted smoothly to afford the corresponding cyclobutenes in good yields ( 3ia–3ka ). Furthermore, the reaction of alkyne 1l bearing a cyclopropyl group gave 3la in 67% yield with the cyclopropyl ring intact. Fig. 2: Scope of the intermolecular reaction. Unless noted otherwise, all reactions were conducted with 0.1 mmol scale under irradiation of 12 W blue LED strip and Ar atmosphere; Isolated yields; Racemates for all cyclobutenes. a Reaction time: 1–18 h. b Reaction time: 24–48 h. c Reaction time: 53 h–3d. d Isolated as N -benzylamide by in-situ treatment with benzylamine after completion of the cycloaddition; Two-step yield. e Reaction time: 5d; the reaction was conducted with 15 equiv. of alkene and PC III instead of PC I . Full size image In addition to the aryl substitution, alkynes substituted with alkyl groups were also examined. We were pleased to find that the reaction with dialkylalkynes 1m and 1n proceeded to afford the corresponding cyclobutenes 3ma and 3na . Moreover, both silyl-substituted and terminal alkynes 1o – 1u smoothly participated in the reaction. We were also intrigued whether the reaction would tolerate substrates with free hydroxyl and carboxylic acid groups, which would allow obviating protecting group chemistry. Indeed, the alkynes 1s and 1u gave cyclobutenes 3si and 3ua in 85 and 78% yield, respectively. 1,3-Diyne 1v turned out to be a good substrate to afford the corresponding alkyne-substituted cyclobutene 3va in 70% yield. Next, we investigated the reactivity of the alkene counterpart, and found that alkenes flanked by electron-withdrawing groups are required for efficient conversion. Thus, those flanked by the functionalities including anhydride, amide, ester, and nitrile participated smoothly in the reaction (Fig. 2 , 3ab – 3cg ). To examine the detailed electronic and steric impact of maleimide on the cycloaddition, various N -substituted maleimides were subjected to the standard conditions. It turned out that both N-H, N -alkyl maleimides 2h and 2i gave the corresponding cyclobutenes 3ah and 3ai in excellent yields. Various N -substituted maleimides including N -benzyloxy, 4-cyanophenyl, and 4-carbomethoxyphenyl maleimides were tolerated to afford cyclobutenes in good to moderate yields ( 3aj – 3al ). In addition, the introduction of N-heteroarenes in the cycloadduct was achieved with the maleimide 2n . The effect of the substitution on the olefinic moiety of maleimide was further investigated. The maleimides 2o – 2r bearing bromo, methoxy, and methyl substituents gave the cyclobutenes in excellent yields. Dimethyl substituted maleimide 2s , however, afforded the corresponding cycloadduct in 55% yield presumably owing to the steric hindrance. Reaction of 2t derived from L -alanine successfully proceeded to give 3at in 93% yield. Whereas acyclic alkenes of mono-activation such as cinnamate failed to give the corresponding cyclobutene ( 3au , see Supplementary Fig. 1 a for unreactive alkenes), cyclic mono-activated alkenes including lactam 3av and lactones ( 3aw – 3xw ) afforded the corresponding products in good to moderate yields. Moreover, a highly sterically hindered product bearing a quaternary center such as 3ax was produced in high yield (76%). We speculate that the failure of the acyclic alkenes may be attributed to the catalyst quenching owing to the pathway involving E / Z isomerization [36] , [37] , [38] . Meanwhile, the observed reactivity of 1a with 2w was compared with that under direct UV-irradiation. It turned out that the reaction was sluggish under both 254 nm and 365 nm (17 and 3%, respectively; see Supplementary Fig. 1b ). Also, late stage modification of commercial drugs containing alkynes proceeded smoothly when performed on O -acetyl 17α-ethynylestradiol and Efavirenz to afford 3ya and 3za in 66 and 45% yield, respectively. A successful implementation of intramolecular alkyne–alkene cycloaddition would offer an access to valuable cyclic compounds. When the ester-tethered enyne 4a was subjected to the optimized reaction conditions, coumarin 6a was obtained in 73% yield ( E / Z = 1:1) (Fig. 3 ). While the formation of diene 6a was unexpected, we speculated that ring opening of the initial cyclobutene accounts for the diene formation. Also, the control experiments without light or photocatalyst showed no reaction (see Supplementary Fig. 2a ). Thus, the photocatalyzed intramolecular enyne cycloaddition allows an access to highly substituted 1,3-dienes readily built from simple enyne substrates, which serves as a complementary means to the enyne metathesis. Interestingly, among the ample literature precedents, the syntheses of these highly substituted 1,3-dienes based on enyne metathesis are scarce with necessitating terminal alkenes. As such, a comparison was performed by using 4a (see Supplementary Fig. 2b ). Whereas the [2 + 2] cycloaddition gave 6a in 73% yield, enyne metathesis failed to give 6a . Fig. 3: Scope of the intramolecular reaction. Unless noted otherwise, all reactions were conducted in 0.1 mmol scale under irradiation of 12 W blue LED strip and Ar atmosphere; Isolated yields. a Reaction time: 1–18 h. b Reaction time: 24–48 h. c Reaction time: 60 h, racemate for 5r . d Reaction was conducted with 0.05 mmol scale; Reaction concentration: 0.01 M. Full size image The examination of the scope of the alkyne substituents revealed broad tolerability (Fig. 3 ). Those substituted with aryl and TMS groups gave the corresponding coumarins in good yields ( 6a and 6b ). Likewise, 2-quinolones 6c – 6e could be synthesized in good to excellent yields by employing amido tethers. Alkynes substituted with various types of substituents including aryl, heteroaryl, and alkyl groups reacted smoothly to give the corresponding 2-quinolones. For example, heteroaryl-substituted 2-quinolones 6f and 6g were readily prepared by employing alkynes bearing pyridine and isoquinoline groups, respectively. Also, substitution of the alkene moiety with various groups including pyridine, furan, ester, and amide was well tolerated ( 6i – 6l ). The effect of steric hindrance on the alkene moiety was examined with the substrate 4m bearing a trisubstituted alkene, which gave 6m in albeit moderate yield. In addition to amido tethers, sulfonamide also turned out to be an effective tether providing a cyclic sulfonamide 6n . Lastly, we examined the feasibility of 5-membered ring formation with ester and amido-tethered substrates afforded the corresponding unsaturated lactone 6o and lactam 6p in 70 and 60%, respectively. Interestingly, the reaction with 4q furnished 6q′ via electrocyclization of the corresponding diene. When silyl-tethered 4r was subjected to the reaction conditions, cyclobutene-fused 7-membered ring product 5r was obtained in 62% yield. Synthetic applications Extended π-systems are an important feature in various applications including fluorescence sensors and material science [59] , [60] , [61] , [62] . As such, we explored the accessibility to such systems based on our synthetic method (Fig. 4a, b ). When we performed an intramolecular [2 + 2] cycloaddition with enyne 4s containing benzofuran as an alkene counterpart, an unexpected product was obtained in 74%, whose structure was assigned as 5s′ (see Supplementary Figs. 346 and 347 ). This is in contrast to the diene formation observed in other intramolecular enynes lacking heterocyclic substituents, which arises from the ring opening of cyclobutenes. The rearrangement could be explained by that excitation of the cyclobutene intermediate 5s leads to the formation of 1,2-diradical I , which undergoes fragmentation to give 1,5-diradical II followed by recombination to give 5s′ . This rearrangement turned out to be quite general in that the benzothiophene derivatives 4t and 4u afforded 5t′ and 5u′ in 99 and 76%, respectively. Fig. 4: Synthesis of extended π-systems and synthetic applications. Racemates for all cyclobutenes. a Tandem cycloaddition followed by rearrangement of benzofuran and benzothiophenes. (ISC = Intersystem crossing). 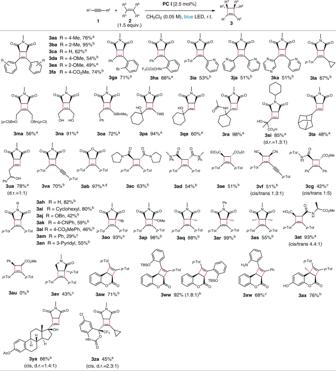Fig. 2: Scope of the intermolecular reaction. Unless noted otherwise, all reactions were conducted with 0.1 mmol scale under irradiation of 12 W blue LED strip and Ar atmosphere; Isolated yields; Racemates for all cyclobutenes.aReaction time: 1–18 h.bReaction time: 24–48 h.cReaction time: 53 h–3d.dIsolated asN-benzylamide by in-situ treatment with benzylamine after completion of the cycloaddition; Two-step yield.eReaction time: 5d; the reaction was conducted with 15 equiv. of alkene andPC IIIinstead ofPC I. b Derivatization of coumarin. (DDQ = 2,3-dichloro-5,6-dicyano-1,4-benzoquinone). c Synthesis of exomethylene cyclobutene. d Synthesis of γ-lactam and pyrrolidine derivatives. Full size image To promote ring expansion, 5t′ was heated at 100 °C. Gratifyingly, tetracyclic compound 6t′ was obtained in 65% yield, which could be rationalized by the thermal electrocyclic ring opening followed by sulfur extrusion. Also, the ring expansion reaction with 5u′ proceeded well to give the rearrangement product 6u′ in 86% yield upon thermolysis. Also, we showed that different phenanthrenes 6a′ and 6a″ could be readily prepared from 6a by oxidative cyclization and benzyne cycloaddition, respectively. The synthetic utility of cyclobutenes were further illustrated by the several transformations (Fig. 4c, d ). Exomethylene cyclobutane 7 was prepared from allylic alcohol 3qa by Johnson-Claisen rearrangement. In addition, 2-pyrrolidone and pyrrolidine could be synthesized in good yields by the reduction of cyclobutenes 3aa and 3ca bearing maleimide. Mechanistic studies To determine whether the reaction involves a radical chain mechanism, we performed light on-off experiments on both inter- and intra-molecular reactions ( 3ca and 6d , respectively, see Supplementary Fig. 4 ). Conversions stopped in the absence of light in both experiments, which rules out a radical chain mechanism. This result was further confirmed by measuring the quantum yield of the cycloaddition of 1a and 2a . The value of 0.91 strongly supports that the cycloaddition is a non-chain reaction (see Supplementary Discussion ). To further corroborate that the EnT process is operative in the cycloaddition, we performed an experiment in the presence of triplet quencher benzil ( E T = 53.4 kcal/mol), and found that the yield significantly decreased to 30%. (Fig. 5a ). Fig. 5: Mechanistic studies. a Effect of triplet quencher. b Stern–Volmer luminescence quenching experiments using a 0.1 mM solution of PC I and variable concentrations of substrate 1m and 2a in CH 2 Cl 2 . Full size image Next, Stern–Volmer quenching experiments on several catalysts were performed by employing 1a and 2a as the quenchers to examine the correlation between the extent of quenching and triplet energy or redox potential (see Supplementary Figs. 7 – 9 ). The degree of quenching among the catalysts by 1a was in good agreement with their triplet energies, not with their redox potentials, in which PC I with the highest triplet energy displays the most significant quenching. Likewise, the same propensity was observed with 2a , albeit the extent of quenching was less efficient compared to 1a . These results suggest that the cycloaddition is promoted via EnT. An ensuing question was which counterpart between the alkyne and alkene undergoes productive triplet excitation, given their similar triplet energies ( 1a 56.7 kcal/mol vs. 2a 55.9 kcal/mol). The analysis of the Stern–Volmer experiments indicates that 1a is a much more efficient quencher compared to 2a , which may suggest that alkynes excited to the triplet state react with the ground state alkenes. On the contrary, no queching of PC I by alkyne 1m was observed, which possesses much higher triplet energy ( E T = 74.1 kcal/mol) than that of PC I , and yet the reaction with 2a provides cyclobutene 3ma in 56% (Fig. 5b ), which leaves only one possibility of the participation of the triplet alkene. To further support the rationale, we performed radical clock experiments (Fig. 6 ). Thus, alkyne 1l and maleimide 2y bearing a cyclopropyl group were prepared, and each of the substrates was reacted with 2a and 1a , respectively (Fig. 6a, b ). Whereas the reaction of cyclopropyl alkyne 1l with maleimide 2a proceeded to give the corresponding cycloadduct 3la in 67% yield, the formation of the isomerization product 2y′ along with cycloadduct 3ay was obtained in low yields when cyclopropyl maleimide 2y was reacted with alkyne 1a . Furthermore, when cyclopropyl maleimide 2y alone was subjected to the reaction conditions, 2y′ was obtained in 73% yield (Fig. 6c ). On the other hand, cyclopropyl alkyne 1l was fully recovered when subjected to the conditions. These results that 2y undergoes ring opening upon excitation while 1l in its triplet state remains intact could be reasoned by the lack of the radical characters at the α-cyclopropyl-substitued carbon in the triplet state 1l . (It was reported that the rate constant for the ring opening of α-(2-phenylcyclopropyl)vinyl radicals is substantially higher than that of the corresponding α-(2-phenylcyclopropyl)carbinyl radical ((1.6 ± 0.2) × 10 10 s −1 and 9.4 × 10 7 s −1 , respectively)) [63] , [64] . Fig. 6: Radical clock experiments. Racemates for all products. a Intermolecular reaction between cyclopropyl alkyne 1l and 2a . b Intermolecular reaction between 1a and cyclopropyl alkene 2y . c Individual reactivity of 2y and 1l under the standard conditions. Full size image To address the question, we performed DFT calculations on Mulliken spin density distributions (Fig. 7a ). Whereas significantly low spin densities on the sp carbons of alkynes 1a (0.251 and 0.251) and 1l (− 0.051 and 0.486) were observed, maleimides 2a and 2y showed much more localized spin densities on the carbons undergoing bond formation (0.778 and 0.774, 0.785 and 0.487, respectively). Fig. 7: Mulliken spin densities (T 1 ) and triplet-singlet energy gaps of selected substrates. a Reactions were conducted with the standard condition using di( p -tolyl)acetylene 1a (0.1 mmol). a Spin densities and surfaces of 1a and 2a ; Spin densities of cyclopropyl derivatives 1l and 2y . b Correlation of spin densities and reaction efficiencies of N -substituted maleimides. Full size image Moreover, during the survey for the scope of maleimides, we observed a wide spread in yields depending on the N-substitution. This prompted us to gauge the correlation between spin density and reaction efficiency (Fig. 7b ). A clear correlation was observed; generally, N -aryl maleimides gave lower yields compared to N -alkyl maleimides, for which the low spin density on the olefinic carbons appears to be responsible. On the other hand, maleimides substituted with electron-deficient aryl groups afforded higher yields, which is also consistent with their spin densities. Based on these experimental and computational studies, we propose that although both alkynes and alkenes undergo triplet excitation, the excited state alkenes react with the ground state alkynes to give the cycloadducts. To examine whether the intramolecular reaction also proceeds via EnT mechanism, we performed a comparison with several photocatalysts. PC II and VI were chosen based on their triplet energies that are similar to or higher than that of 4c (49.0 kcal/mol). As a control, those with lower triplet energies, Ru(bpy) 3 (PF 6 ) 2 and Eosin Y, were also included. As shown in Fig. 8 , the results were consistent with the triplet energies of the catalysts. Moreover, it is noteworthy that PC VI , which was ineffective in the intermolecular reaction owing to the low triplet level relative to the maleimide (55.9 kcal/mol), provided 6c in 67%. Also, we investigated the redox property of 4c with cyclic voltammetry (see Supplementary Fig. 11 ), the low reduction potential ( E p/2 red = −2.13, −2.44 V vs SCE) of which makes it unlikely to undergo reduction by the catalysts examined. Likewise, oxidative pathway could be ruled out based on the oxidation potentials of the catalysts. These results indicate that EnT mechanism is responsible for the intramolecular cycloaddition. Fig. 8: Comparison of selected photocatalysts. Reactions were performed with 0.025 mmol scale under Ar. Yields determined by 1 H NMR spectroscopic analysis against an internal standard. (1,1,2-trichloroethene). a Green LED was used instead of blue LED. Full size image To shed light on the reaction pathway, we performed DFT calculations on the intermolecular and intramolecular reaction pathways. All calculations were carried out with the Gaussian 09 software [65] using the M06 functional [66] with the 6-311 + g(d,p) basis set [67] , [68] . The SMD solvation model [69] with the solvent of dichloromethane (ε = 8.93) was used for all calculations. The DFT calculations on the intermolecular cycloaddition between alkyne 1a and maleimide 2a revealed that excitation of 2a to its T 1 state (55.9 kcal/mol) by the catalyst followed by the reaction with alkyne 1a leads to the formation of the triplet intermediate Int-3aa via TS-3aa (ΔG ‡ = 7.2 kcal/mol) (Fig. 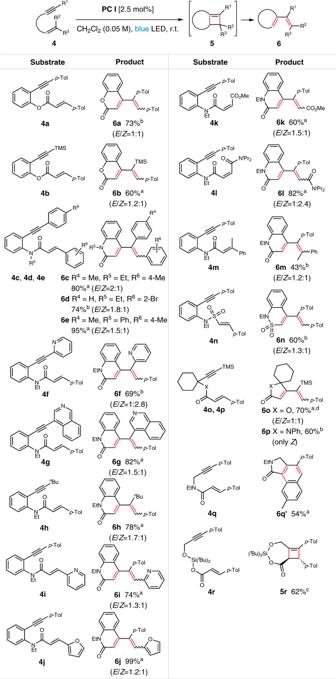Fig. 3: Scope of the intramolecular reaction. Unless noted otherwise, all reactions were conducted in 0.1 mmol scale under irradiation of 12 W blue LED strip and Ar atmosphere; Isolated yields.aReaction time: 1–18 h.bReaction time: 24–48 h.cReaction time: 60 h, racemate for5r.dReaction was conducted with 0.05 mmol scale; Reaction concentration: 0.01 M. 9a ). Subsequently, conversion to open-shell singlet state Int-3aa′ allows the formation of cyclobutene 3aa via barrierless TS-3aa′ . On the other hand, we were intrigued by the formation of 1,3-dienes instead of cyclobutenes from the intramolecular reaction. Our hypothesis was that tandem triplet activation of the initial cyclobutenes may account for the formation of 1,3-dienes. Thus, we performed DFT calculations on the reaction pathway involving the formation of 1,3-dienes via cyclobutenes as intermediates, and compared the activation barrier with that of thermal electrocyclic ring opening (Fig. 9b, c ). The formation of cyclobutene 5c is initiated by the excitation of 4c to its triplet state (49.0 kcal/mol) by the catalyst. The addition to the alkyne to form triplet diradical Int-5c via TS-4c (ΔG ‡ = 5.9 kcal/mol) followed by conversion to the open-shell singlet state Int-5c′ via barrierless TS-5c results in the formation of cyclobutene 5c . Fig. 9: DFT calculations. a Intermolecular cycloaddition between alkyne 1a and maleimide 2a . b Formation of putative cyclobutene intermediate 5c from the intramolecular reaction of 4c . c Formation of 1,3-dienes from 5c . Full size image It turns out that cyclobutene 5c could be readily excited to its T 1 state (41.2 kcal/mol) by the catalyst (60.8 kcal/mol for T 1 state) (Fig. 9c ). Rearrangement of the triplet diradical affords Int-6ca / 6cb with the activation barrier of 15.5 kcal/mol, which results in the formation of diene 6ca / 6cb . In comparison, the activation barrier of the thermal electrocyclic ring opening via TS-6c′ turned out to be significantly higher (21.2 kcal/mol). These results are in contrast to the cyclobutenes derived from intermolecular cycloaddition, in which a significantly higher ΔG ‡ (29.5 kcal/mol) appears to be responsible for interrupting ring opening (see Supplementary Fig. 12 ). We developed alkyne–alkene [2 + 2] cycloaddition based on visible light EnT photocatalysis. Whereas the formation of cyclobutenes was observed from intermolecular reactions, 1,3-dienes were obtained from intramolecular reactions. For the intermolecular cycloaddition, a broad range of alkynes reacted smoothly with electron-deficient alkenes to afford the corresponding cyclobutenes. On the other hand, for the 1,3-diene formation in the intramolecular reactions, the ring opening of cyclobutene intermediates via tandem triplet excitation is responsible. Synthetically, the [2 + 2] enyne cycloaddition offers a complementary means to the Ru(II)-catalyzed enyne metathesis for the synthesis of highly substituted 1,3-dienes. Various experimental evidences support that between the two reactants, alkyne and alkene, the alkene undergoes productive excitation to a triplet state to react with the ground state alkyne. We also demonstrated the utility of the method including the synthesis of various extended π-system. General procedure for the synthesis of cyclobutenes Alkyne (0.1 mmol, 1.0 equiv. 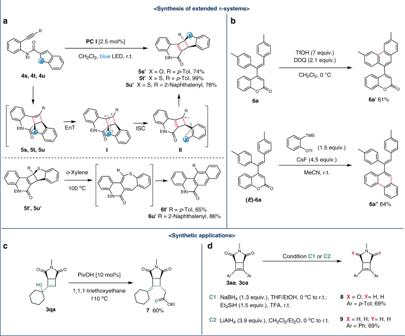Fig. 4: Synthesis of extended π-systems and synthetic applications. Racemates for all cyclobutenes.aTandem cycloaddition followed by rearrangement of benzofuran and benzothiophenes. (ISC = Intersystem crossing).bDerivatization of coumarin. (DDQ = 2,3-dichloro-5,6-dicyano-1,4-benzoquinone).cSynthesis of exomethylene cyclobutene.dSynthesis of γ-lactam and pyrrolidine derivatives. ), alkene (1.5 equiv. ), and photocatalyst Ir[dF(CF 3 )ppy] 2 (dtbbpy)PF 6 ( PC I , 2.5 mol%) were added to an oven-dried 4 mL vial equipped with a stir bar. 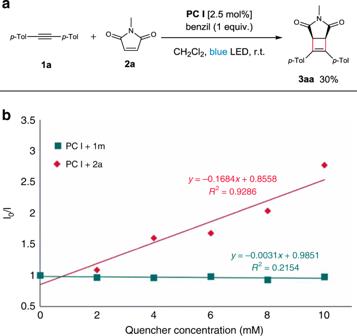Fig. 5: Mechanistic studies. aEffect of triplet quencher.bStern–Volmer luminescence quenching experiments using a 0.1 mM solution ofPC Iand variable concentrations of substrate1mand2ain CH2Cl2. 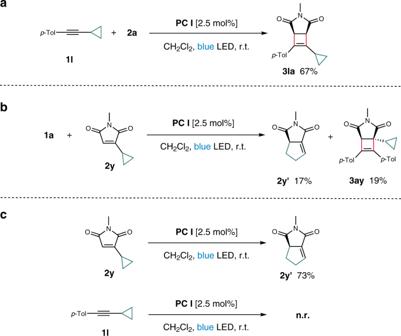Fig. 6: Radical clock experiments. Racemates for all products.aIntermolecular reaction between cyclopropyl alkyne1land2a.bIntermolecular reaction between1aand cyclopropyl alkene2y.cIndividual reactivity of2yand1lunder the standard conditions. 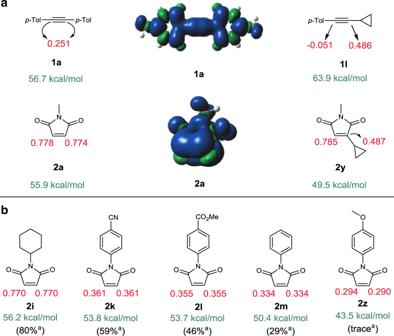Fig. 7: Mulliken spin densities (T1) and triplet-singlet energy gaps of selected substrates. aReactions were conducted with the standard condition using di(p-tolyl)acetylene1a(0.1 mmol).aSpin densities and surfaces of1aand2a; Spin densities of cyclopropyl derivatives1land2y.bCorrelation of spin densities and reaction efficiencies ofN-substituted maleimides. The combined materials were dissolved in CH 2 Cl 2 (2 mL) under argon atmosphere in glovebox. The reaction mixture was then irradiated by 12 W blue LED strip at room temperature (maintained with a cooling fan). 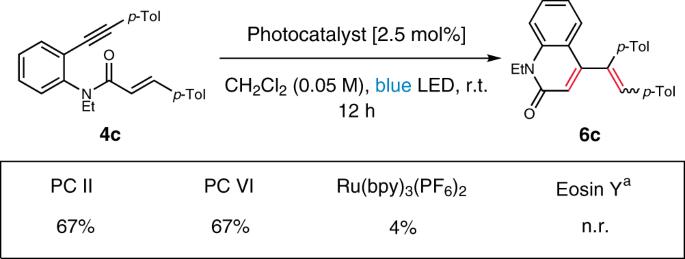Fig. 8: Comparison of selected photocatalysts. Reactions were performed with 0.025 mmol scale under Ar. Yields determined by1H NMR spectroscopic analysis against an internal standard. (1,1,2-trichloroethene).aGreen LED was used instead of blue LED. 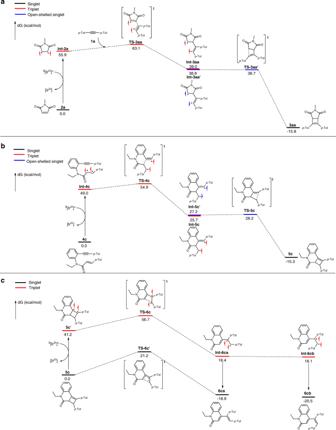Fig. 9: DFT calculations. aIntermolecular cycloaddition between alkyne1aand maleimide2a.bFormation of putative cyclobutene intermediate5cfrom the intramolecular reaction of4c.cFormation of 1,3-dienes from5c. After completion of the reaction as indicated by TLC, the solution was concentrated under reduced pressure. The residue was purified by flash column chromatography on silica gel to give the desired product. See Supplementary Methods for further experimental details.